Room temperature high-fidelity holonomic single-qubit gate on a solid-state spin At its most fundamental level, circuit-based quantum computation relies on the application of controlled phase shift operations on quantum registers. While these operations are generally compromised by noise and imperfections, quantum gates based on geometric phase shifts can provide intrinsically fault-tolerant quantum computing. Here we demonstrate the high-fidelity realization of a recently proposed fast (non-adiabatic) and universal (non-Abelian) holonomic single-qubit gate, using an individual solid-state spin qubit under ambient conditions. This fault-tolerant quantum gate provides an elegant means for achieving the fidelity threshold indispensable for implementing quantum error correction protocols. Since we employ a spin qubit associated with a nitrogen-vacancy colour centre in diamond, this system is based on integrable and scalable hardware exhibiting strong analogy to current silicon technology. This quantum gate realization is a promising step towards viable, fault-tolerant quantum computing under ambient conditions. Quantum gates based on geometric phase shifts [1] are a promising resource for intrinsically fault-tolerant quantum computing [2] . While initial proposals for geometric quantum computing [2] based on non-Abelian, adiabatic holonomies [3] entailed slow gate speeds and were thus prone to decoherence, fast schemes [4] employing Abelian, non-adiabatic phases [5] lacked computational universality. Recently, a scheme for non-adiabatic, non-Abelian holonomic quantum computation has been proposed [6] . While the non-Abelian nature of this gate provides computational universality [2] , [7] , the fact that it is non-adiabatic allows for fast quantum gate operation, high clock frequencies and thus intrinsic protection against decoherence. The superior robustness of this quantum gate against decay, dephasing and parametric imperfections (as for example absolute and relative detuning and pulse errors) has been confirmed analytically and by comprehensive numerical simulations [6] , [8] . Originally, the proposal for this holonomic quantum gate [6] was given for a three-level Λ-type system, where the computational basis states are the mutually uncoupled two lower states, while the upper state acts as an ancilla and remains unpopulated before and after the gate operation. A single-qubit gate based on this scheme [6] was recently demonstrated on a transmon qubit [9] , but this approach is limited to cryogenic temperatures; another holonomic quantum computing realization on a room temperature liquid nuclear magnetic resonance system [10] is fundamentally challenged by difficulties to initialize nuclear magnetic resonance systems into pure states. Here we demonstrate a high-fidelity realization of this holonomic single-qubit gate using an individual solid-state spin qubit under ambient conditions. By selecting the electron spin of a nitrogen-vacancy (NV) centre in diamond to create holonomic quantum gates at room temperature, we choose a quantum computing architecture that is based on integrable [11] and scalable [12] solid-state hardware exhibiting strong analogy to current state-of-the-art silicon technology. In our demonstration we achieve close to perfect process fidelities that comply with the error threshold requirement for the implementation of certain fault-tolerant quantum computing protocols [13] . This realization is a promising step towards viable quantum computing at room temperature. NV centre in diamond The negatively charged NV centre in diamond holds great promise for quantum sensing [14] , [15] , [16] and quantum information applications [17] , [18] . NV electron spins stand out as potential room temperature qubits, because they can be manipulated on the nanosecond time scale [19] while featuring coherence times of milliseconds under ambient conditions [20] . Both initialization [21] , [22] and read-out [18] of the NV electron spin, as well as dynamic single-qubit gates [23] and dynamic entanglement generation of two coupled NV centres [24] have been demonstrated. First implementations of quantum algorithms were reported recently [25] . As the NV centre fulfils the DiVincenzo criteria for quantum computers remarkably well, the realization of an NV centre based quantum computer ultimately depends on the achievable fidelities of elementary quantum gates. While quantum error correction codes have been proposed [26] , they will be applicable only if the fidelity of each elementary gate exceeds a certain threshold. Reaching this threshold [13] , (single gate error rates are predicted to range between 10 −6 and 10 −2 ) requires resorting to a hardware that is intrinsically fault-tolerant. To this end, hardware based on geometric phases and decoherence-free subspaces are particularly promising. For negligible hyperfine coupling and strain, the Hamiltonian of the ground state triplet of the NV centre is defined by the zero-field splitting D =2 π × 2.87 GHz and the Zeeman splitting with the external magnetic field B , electron gyromagnetic ratio γ e and the electron spin S . The NV electron spin forms a V-type three-level scheme (cf. Fig. 1c ) made up of the m s =0 and m s =±1 levels (denoted by |0›, |+› and |−› in the following). At an external magnetic field of | B |≈404 G, the transitions |0›↔|+› at ω 0+ =2π × 4.003 GHz and |0›↔ |−› at ω 0− =2π × 1.738 GHz can be driven coherently by microwave radiation at frequencies ω + = ω 0+ + δ + and ω − = ω 0− + δ − , respectively. 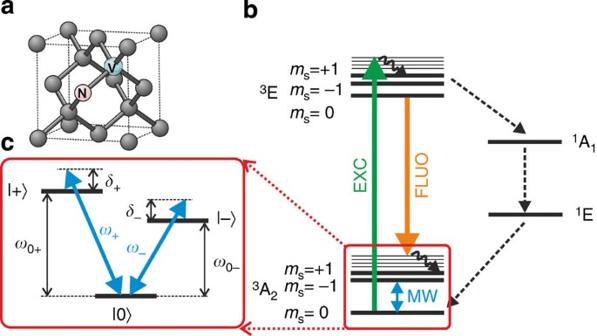Figure 1: NV centre geometry and level structure. (a) Illustration of the unit cell of diamond including an NV colour centre. Spin projectionsms=0,±1 are defined with respect to the NV symmetry axis. (b) Energy levels of the triplet (left) and singlet states (right) of the NV centre and the applied excitation (EXC) and microwave (MW) fields and the detected fluorescence (FLUO). (c) Three-level V-scheme of the NV ground state triplet employed for the realization of the single-qubit holonomic quantum gate. Figure 1b displays the NV level scheme indicating the optical transitions used for spin initialization and readout along with the applied microwave field transitions. Figure 1: NV centre geometry and level structure. ( a ) Illustration of the unit cell of diamond including an NV colour centre. Spin projections m s =0,±1 are defined with respect to the NV symmetry axis. ( b ) Energy levels of the triplet (left) and singlet states (right) of the NV centre and the applied excitation (EXC) and microwave (MW) fields and the detected fluorescence (FLUO). ( c ) Three-level V-scheme of the NV ground state triplet employed for the realization of the single-qubit holonomic quantum gate. Full size image Holonomic single-qubit quantum gate The holonomic quantum gate [6] is defined on a three-dimensional Hilbert space 3 .The computational basis states, here |+› and |−›, span a two-dimensional subspace 2 of that total space. The holonomic quantum gate is carried out by a transformation of the subspace 2 along a smooth, closed loop :[0, T ] t ↦ 2 ( t ), such that 2 (0)= 2 ( T ) (see illustration in Fig. 2a ). For the duration of the holonomic transformation, the |0› state acts as an idle ancilla that stays unoccupied before and after the quantum gate acts. 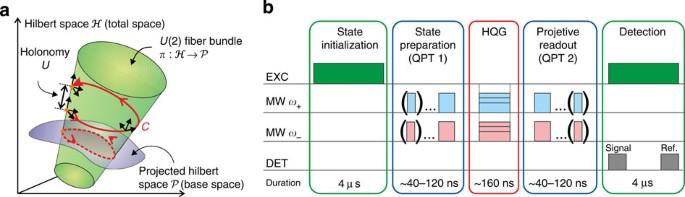Figure 2: Concept for the realization of an NV-based holonomic single-qubit gate. (a) Schematic representation of the total Hilbert space and a projected Hilbert space therein defined through a projective map π:↦by means of the localU(2) fibre bundle. Driving the system on a suitable loop (red curve) on thisU(2) fibre bundle of nontrivial topology gives rise to a holonomy. Here, this holonomy is employed for the generation of a relative phase for quantum computation applications. (b) Experimental sequence for the quantum process tomography (QPT): First the NV state is initialized by a green laser pulse (EXC) to state |0›. In the following first part of the QPT microwave pulses (MW) tuned toω+andω−prepare the spin into one of the nine QPT states |ψj›. After application of the holonomic quantum gate (HQG), the second part of the QPT project the NV state onto one of the nine measurement bases |ψj› by means of microwave pulses (MW). State selective detection concludes the sequence composed of simultaneous application of a green laser pulse (EXC) and signal and reference windows detection (DET). Due to the different numbers and types of pulses necessary for the 81 preparation and readout combinations of the QPT, the durations of the QPT blocks 1 and 2 vary for each QPT measurement. In the rotating frame the NV interaction Hamiltonian reads Figure 2: Concept for the realization of an NV-based holonomic single-qubit gate. ( a ) Schematic representation of the total Hilbert space and a projected Hilbert space therein defined through a projective map π: ↦ by means of the local U (2) fibre bundle. Driving the system on a suitable loop (red curve) on this U (2) fibre bundle of nontrivial topology gives rise to a holonomy. Here, this holonomy is employed for the generation of a relative phase for quantum computation applications. ( b ) Experimental sequence for the quantum process tomography (QPT): First the NV state is initialized by a green laser pulse (EXC) to state |0›. In the following first part of the QPT microwave pulses (MW) tuned to ω + and ω − prepare the spin into one of the nine QPT states | ψ j ›. After application of the holonomic quantum gate (HQG), the second part of the QPT project the NV state onto one of the nine measurement bases | ψ j › by means of microwave pulses (MW). State selective detection concludes the sequence composed of simultaneous application of a green laser pulse (EXC) and signal and reference windows detection (DET). Due to the different numbers and types of pulses necessary for the 81 preparation and readout combinations of the QPT, the durations of the QPT blocks 1 and 2 vary for each QPT measurement. Full size image where the holonomic transformation is carried out through the application of two resonant ( δ + = δ − =0) controlled microwave pulses simultaneously driving the |0›↔ |+› and |0›↔ |−› spin transitions with Rabi frequencies Ω ( t ) γ + and Ω ( t ) γ − , respectively and featuring a joint pulse envelope Ω ( t ). To provide a cyclic state evolution, the transformation needs to satisfy and the Rabi weights γ + and γ − need to be properly normalized: | γ + |+| γ − |=1. To ensure the parallel transport condition for a purely geometric evolution ‹ ψ k | H int | ψ j ›= δ jk the ratio of the Rabi frequencies has to be kept constant. In this case the dressed system undergoes a Rabi oscillation between the bright state and the excited state | e ›=|0›, whereas the dark state | d ›= − γ − |+›+ γ + |−›) is decoupled from the dynamics. In compliance with the aforementioned conditions, the characteristic structure of the Hamiltonian H int ( t ) gives rise to a nontrivial topology of the subspace 2 in the total space 3 and drives the holonomic transformation of the computational states where the Rabi frequency weights can be parameterized by two angles θ and φ as γ + = e iφ sin( θ /2) and γ − =−cos( θ /2). Hence, the complex valued Rabi frequency ratio γ + / γ − determines the kind of quantum gate by choosing a specific set of θ and φ defining a characteristic path ( θ , φ ) on the Grassmannian manifold (3;2). In Table 1 , we list the respective parameter sets ( θ , φ , γ + γ − ) defining some elementary single-qubit quantum gates: the Pauli-X (bit flip gate), Pauli-Y (bit+phase flip gate), Pauli-Z (phase flip gate) and the Hadamard gate. We determine the fidelity of the conducted holonomic quantum gates by performing standard quantum process tomography (QPT) [27] . 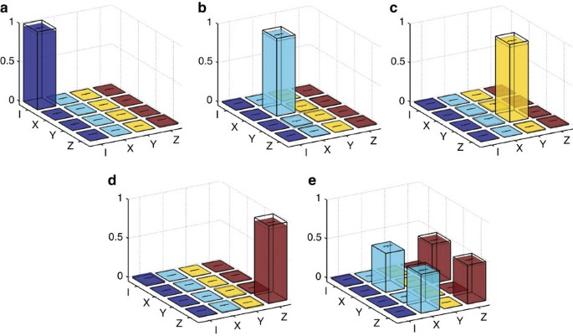Figure 3: Representations of the experimentally accomplished quantum processes. (a) Process matrix of the identity operation, (b) the Pauli-X, (c) the Pauli-Y, (d) the Pauli-Z and (e) the Hadamard gate (coloured bars: experimental data and and error bars, transparent boxes: ideal quantum gates). Figure 3 displays the real parts of the experimentally achieved quantum gate process matrices (coloured bars; imaginary parts are smaller than the respective errors) versus the ideal quantum gates (hollow frame bars). For all three Pauli gates and the Hadamard gate, we achieved total process fidelities around F =0.98 (see Table 2 ) when we apply standard QPT. Note that the QPT, that is, the state preparation before and projective readout after the quantum gate, represents the major part of the experimental sequence (see Fig. 2b ). As it is performed through microwave-induced dynamical phase shifts, the QPT is more prone to noise, parameter imperfection and decoherence effects than our holonomic quantum gate. Since the QPT is not part of the quantum gate, it is instructive to assess the corrected fidelities of the i -th holonomic quantum gate after gauging with the fidelity F Id of a QPT executed without quantum gate (that is, with that of the identity operation). Thereby, we obtain fidelities of the holonomic quantum gates around (see Table 2 ), thus entering the fidelity regime where advanced quantum error correction techniques can become efficacious. Note, that the fidelities reported here were achieved without any of the commonly used post-selection [28] which, if applied, could increase the fidelity of the demonstrated holonomic quantum gates even further. Table 1 Theoretical and experimental parameter settings. Full size table Figure 3: Representations of the experimentally accomplished quantum processes. ( a ) Process matrix of the identity operation, ( b ) the Pauli-X, ( c ) the Pauli-Y, ( d ) the Pauli-Z and ( e ) the Hadamard gate (coloured bars: experimental data and and error bars, transparent boxes: ideal quantum gates). Full size image Table 2 Experimentally achieved fidelities. Full size table Altogether, we showed that NV centre electron spins in diamond enable the realization of high-fidelity, non-adiabatic, non-Abelian holonomic single-qubit gates at room temperature. Acting on the NV electron spin, this quantum gate is directly compatible with recently developed techniques employing coupling to proximal nuclear spins (such as those provided by 13 C nuclei or the NV’s own 14 N/ 15 N spin), for example, for temporary qubit storage (quantum memory). However, contrary to other demonstrations employing the NV electron spin primarily as a mediator for the control of randomly distributed proximal nuclear spin qubits, our technique allows for the controlled design of a truly engineered quantum computing architecture based on NV electron spins as computational nodes and employing the built-in NV nitrogen nucleus as a quantum memory. For universal holonomic quantum computation, the single-qubit gate presented here needs to be combined with a holonomic two-qubit gate. To this end, it is straightforward to consider two electron spins of a pair of adjacent NV centres that are coupled by magnetic dipole–dipole interaction. The far-field optical addressing and readout of individual NV spins could be achieved using the diffraction-unlimited resolution provided by stimulated emission depletion microscopy [29] , which is our long-term vision. In combination with optimal control techniques [30] such a universal set of holonomic quantum gates can allow for a truly scalable and fault-tolerant quantum computation architecture based on room temperature solid-state hardware. Moreover, the demonstrated robust high-fidelity holonomic phase gates could be employed for other challenging spin manipulation applications to enhance high-fidelity dynamical decoupling protocols or to allow for robust high-sensitivity quantum sensing. Electron spin manipulation The gate was realized on a naturally occurring NV centre in synthetically grown, electronic grade diamond. For spin initialization and fluorescence readout, the NV centres were optically addressed by a 532 nm continuous wave laser via a home-build confocal microscope. The microwave pulses were synthesized by a Tektronix AWG 7122C, amplified and coupled into a microwave strip line spanned across the diamond sample. Typically the Rabi frequencies were around 6 MHz. The external magnetic field was applied through a permanent magnet and aligned to be parallel to the NV axis to an angle deviation of <2°. The lifetimes of the |+› and |−› states with respect to the |0› were both T 1 =(5±1) ms, while the coherence times of the |+› and |−› states with respect to the |0› state were both μs. By applying a magnetic field of | B |≈404 G, we tuned the NV system near the triplet excited state level anti-crossing, providing us with a polarization of the 14 N nuclear spin into the m I =+1 hyperfine state. Quantum process tomography For the evaluation of the experimentally achieved quantum gates, we conducted standard QPT [27] . An arbitrary operation ε acting on an initial state ρ in and generating the final state ρ out can be described by a quantum process matrix χ mn in terms of a quantum dynamical map , where the E m ε SU ( d ) represent a full set of orthogonal basis operators (here, the Gell-Mann operators as the generators of the SU (3)). The fidelity of the quantum process is then given by the overlap between the experimental and theoretical representation of the process matrix χ exp and χ theo , respectively: F = tr ( χ exp · χ theo ). Here, the QPT is performed in 81 runs, in each of which the system has to be initialized into one of nine (quasi-)pure states | ψ j ›ε(| ψ 1 ›, | ψ 2 ›,…, | ψ 9 ›), where the | ψ j › are chosen such that the corresponding density matrices ρ j =| ψ j ›‹ ψ j | form a basis set for the space of matrices: ρ =∑ j q j | ψ j ›‹ ψ j |. The reconstructed process matrix χ mn was fitted by means of a maximum-likelihood estimation procedure assuming the process matrix to be completely positive and not trace increasing (for details see Supplementary Notes 1–5 ). How to cite this article : Arroyo-Camejo, S. et al . Room temperature high-fidelity holonomic single-qubit gate on a solid-state spin. Nat. Commun. 5:4870 doi: 10.1038/ncomms5870 (2014).